Regulation of miR-200c/141 expression by intergenic DNA-looping and transcriptional read-through The miR-200 family members have been implicated in stress responses and ovarian tumorigenesis. Here, we find that miR-200c/141 transcription is intimately linked to the transcription of the proximal upstream gene PTPN6 (SHP1) in all physiological conditions tested. PTPN6 and miR-200c/141 are transcriptionally co-regulated by two complementary mechanisms. First, a bypass of the regular PTPN6 polyadenylation signal allows the transcription of the downstream miR-200c/141. Second, the promoters of the PTPN6 and miR-200c/141 transcription units physically interact through a 3-dimensional DNA loop and exhibit similar epigenetic regulation. Our findings highlight that transcription of intergenic miRNAs is a novel outcome of transcriptional read-through and reveal a yet unexplored type of DNA loop associating two closely located promoters. These mechanisms have significant relevance in ovarian cancers and stress response, pathophysiological conditions in which miR-200c/141 exert key functions. The miR-200 family consists of five microRNAs (miRNAs: miR-141, 200a, 200b, 200c and 429) located in two intergenic genomic clusters on chromosomes 1 and 12 in humans. Several reports highlighted the impact of the miR-200 in cancer development and progression [1] , [2] , [3] , [4] , [5] , [6] , [7] , [8] , [9] , [10] . The miR-200 family regulates key processes in tumorigenesis, such as epithelial–mesenchymal transition [5] , [11] , [12] , [13] , [14] , [15] , [16] , [17] , migration and invasion [18] , [19] , [20] , stem cell maintenance [6] , [21] , [22] , [23] , stromal remodelling [24] , [25] and oxidative stress response [7] , [26] , [27] , [28] . Moreover, miR-200 expression is induced by oxidative stress in various cells and tissues [7] , [26] , [28] , [29] , [30] , [31] . Finally, these miRNAs accumulate and play a key role in ovarian tumorigenesis and chemosensitivity, the oxidative stress response being one important feature [2] , [4] , [5] , [7] , [9] , [10] , [32] , [33] , [34] , [35] , [36] . Given the important role of miR-200 family members in oxidative stress response and ovarian tumorigenesis, understanding their regulation in these conditions is of major interest. Here we focus on the regulation of the intergenic miR-200 genomic cluster comprising miR-200c and miR-141. Previous studies have identified ZEB1/ZEB2 and p53 transcription factors as regulators of the expression of these miRNAs [11] , [15] , [37] , [38] , [39] . Moreover, epigenetic marks such as DNA and histone methylation have also been linked to miR-200 expression, especially between epithelial and mesenchymal cells [40] , [41] , [42] , [43] . However, despite these efforts, the regulatory mechanisms involved in miR-200 expression are still far from being completely understood. In contrast to intronic miRNAs that are frequently transcribed along with their host genes, it is widely assumed that the regulation of intergenic miRNAs, such as miR-200c and miR-141, relies on their own promoters [44] , [45] . We show here that transcription of intergenic miRNAs can also be modulated by their surrounding genes. Indeed, alternative polyadenylation (APA) and transcriptional read-through of an upstream gene can be new means of producing intergenic miRNAs. APA concerns about half of the human genes. APA shortens or lengthens the 3′-extremity of messenger RNAs and subsequently affects mRNA stability or protein translation [46] . Although it has not yet been described to date, a new outcome for APA could be the transcription of miRNAs located between two alternative polyA sites. Another yet unexplored mechanism that could also participate in the regulation of intergenic miRNA expression is a chromatin interaction between its promoter and another regulatory locus. Recent reports underline the functionality of both long-range and short-range chromatin contacts [47] , [48] , [49] . Short-range DNA loops can bring together the promoter and terminator regions of the same gene. This type of DNA conformation, called ‘gene-loop’, plays a role in transcriptional memory and directionality and has been identified from yeast to mammals [50] . However, the role of such DNA interactions on intergenic miRNA regulation has not been established so far. Here, we show evidence that the miR-200c/141 intergenic cluster is regulated through two original complementary mechanisms: the read-through of the transcription of a neighbouring gene and the three-dimensional (3D) chromatin interaction involving the miRNA promoter region. We demonstrate that the transcription of miR-200c/141 is tightly associated with that of PTPN6 (also called SHP1 ), a gene whose 3′ extremity is located less than 3 kilobases upstream of the miRNAs. We show that the bypass of the usual PTPN6 polyadenylation signal can lead to the transcription of miR-200c/141, and we reveal the existence of a 3D DNA conformation associating the promoters of these two genes. Together, our data indicate a physiological relevance of PTPN6 expression in miR-200c/141 regulation in all tested situations. We propose that the systematic correlation between these two genes in several different contexts is due to transcriptional read-through of the PTPN6 gene and a previously unexplored type of DNA loop associating two closely located promoters. miR-200c and miR-141 are regulated at transcriptional level Regulation of miR-200c and miR-141 (hereafter referred to as miR-200c/141) expression represents a crucial step in ovarian tumorigenesis and stress response. A better understanding of their regulation deserved further investigation in these two related pathophysiological conditions. As both miR-200c and miR-141 are transcribed from the same genomic locus, we first observed that the levels of the two mature miRNAs were directly proportional to their corresponding primary transcript (below referred to as pri-miR-200c-141 ) in the diverse conditions analysed, that is, following acute oxidative stress and in high-grade ovarian carcinomas (HGSOC; Fig. 1a–d and Supplementary Fig. 1a,b ). Indeed, the kinetics of miR-200c/141 accumulation after exposure to H 2 O 2 followed the increase of pri-miR-200c-141 transcript in epithelial or fibroblast cell lines from both human or mouse origin ( Fig. 1a,b and Supplementary Fig. 1a,b ). We detected oxidative stress-mediated miR-200c/141 upregulation in all cell lines tested, except those already expressing high basal concentrations of the miR-200c/141, such as IGROV-1 cell line ( Supplementary Fig. 1d ). Similarly, basal levels of mature and primary miR-200c/141 were found significantly correlated in different ovarian and breast cancer cell lines ( Fig. 1c ) as well as in a cohort of 107 human primary HGSOC ( Fig. 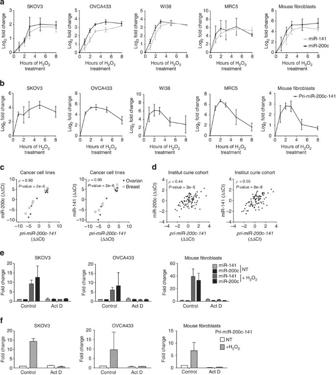Figure 1: Transcriptional regulation is crucial for miR-200c and miR-141 expression. (a,b) Kinetics of accumulation of miR-200c (black) and miR-141 (grey;a) and their corresponding primary transcript,pri-miR-200c-141(b), following H2O2treatment in human ovarian cancer cell lines (SKOV3, OVCA433), human (WI38, MRC5) and mouse fibroblasts, as indicated. qRT–PCR data are means of fold changes (normalized to untreated and expressed as log2)±s.d.n=3 independent experiments at least, except for OVCA433,n=2 (in this case error bars indicate range of data). Kinetics of accumulation in eight other cell lines can be found inSupplementary Fig. 1. Sequences of the pri-miR-200c-141F/R primers from mouse or human origins are given inSupplementary Table 2. (c,d) Scatter plots showing that levels of miR-200c (left) and miR-141 (right) are correlated withpri-miR-200c-141primary transcript levels in ovarian (IGROV-1, OV90, OV2008, OVCAR3, OVCA433, RMG1, SHIN3, SKOV3) and breast (SKBr3, MDA-MB-468, MCF7, MDA-MB-231, MDA-MB-436, MDA-MB-453, BT549) cancer cell lines (c) and in HGSOC (d). qRT–PCR data are shown as normalized cycle threshold centred to the mean (ΔΔCt). Spearman correlation coefficientsρ(rho) and correspondingP-values are indicated on each graph.n=3 independent experiments per cell line, except for OVCAR3 cells,n=2. (e,f) Effect of the transcription inhibitor actinomycin D (Act D) on the levels of miR-141 (grey) or miR-200c (black) (e) and their corresponding primary transcript,pri-miR-200c-141(f), under untreated conditions (NT) or following 3 h of H2O2treatment (+H2O2). Cells were pretreated for 4 h with Act D or dimethylsulphoxide (control). qRT–PCR data are shown as fold change±s.d. of treated compared with untreated cells.n≥2 independent experiments per cell line. 1d and Supplementary Table 1 for description of the cohort). This suggested that the accumulation of miR-200c and miR-141 relies mainly on the regulation of their transcription, rather than on maturation steps. Accordingly, treatment with actinomycin D, an effective transcriptional inhibitor, abolished the increase of miR-200c and miR-141 upon H 2 O 2 exposure ( Fig. 1e,f ). Thus, our data suggest that transcription is a major regulatory step controlling the accumulation of mature miR-200c/141. Figure 1: Transcriptional regulation is crucial for miR-200c and miR-141 expression. ( a , b ) Kinetics of accumulation of miR-200c (black) and miR-141 (grey; a ) and their corresponding primary transcript, pri-miR-200c-141 ( b ), following H 2 O 2 treatment in human ovarian cancer cell lines (SKOV3, OVCA433), human (WI38, MRC5) and mouse fibroblasts, as indicated. qRT–PCR data are means of fold changes (normalized to untreated and expressed as log 2 )±s.d. n =3 independent experiments at least, except for OVCA433, n =2 (in this case error bars indicate range of data). Kinetics of accumulation in eight other cell lines can be found in Supplementary Fig. 1 . 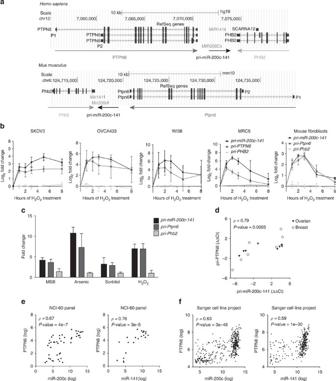Figure 2:pri-miR-200c-141expression correlates withPTPN6transcription. (a) Schematic representation (adapted fromhttp://genome.ucsc.edu) of miR-200c/141 genomic locus showing upstream (PTPN6) and downstream (PHB2, SCARNA12) neighbouring genes in human and mouse species, as indicated. Genomic positions, scale and genome versions used (hg19andmm10) are indicated on the top. Horizontal arrows indicate the sense of transcription. Coding exons are indicated as blocks connected by horizontal lines representing introns, and arrowheads showing sense of transcription. Untranslated regions are presented by thinner blocks. P1 and P2 indicate the alternative promoters used forPTPN6transcription in non-haematopoietic and haematopoietic cells, respectively. (b) Kinetics of accumulation ofpri-miR-200c-141, pri-PTPN6andpri-PHB2primary transcripts following H2O2treatment in human ovarian cancer cells (SKOV3, OVCA433), human (WI38, MRC5) and mouse fibroblasts. qRT–PCR data are means of fold changes (normalized to untreated and expressed as log2)±s.e.m.n=3 independent experiments at least, except for OVCA433,n=2 (in this case error bars indicate range of data). Sequences of the primers from mouse or human origins (pri-miR-200c-141F/R and pri-PTPN6/Ptpn6(2) F/R) used are given inSupplementary Table 2. (c) Effect of different stresses onpri-miR-200c-141, pri-Ptpn6andpri-Phb2primary transcript levels. MSB, menadione sodium bisulfite. qRT–PCR data are shown as fold change±s.d. following treatments, compared with untreated fibroblasts (NT).n=3 independent experiments. (d) Scatter plot showing correlation betweenpri-PTPN6andpri-miR-200c-141primary transcript levels in ovarian and breast cancer cells. qRT–PCR data are shown as normalized cycle threshold centred to the mean (ΔΔCt). (e,f) Scatter plots showing that miR-200c (left) and miR-141 (right) levels are correlated withPTPN6mRNA levels in NCI-60 panel of cell lines (e) and Sanger Cell Line Project (f). Spearman correlation coefficientsρ(rho) andP-values are indicated on each graph. Sequences of the pri-miR-200c-141F/R primers from mouse or human origins are given in Supplementary Table 2 . ( c , d ) Scatter plots showing that levels of miR-200c (left) and miR-141 (right) are correlated with pri-miR-200c-141 primary transcript levels in ovarian (IGROV-1, OV90, OV2008, OVCAR3, OVCA433, RMG1, SHIN3, SKOV3) and breast (SKBr3, MDA-MB-468, MCF7, MDA-MB-231, MDA-MB-436, MDA-MB-453, BT549) cancer cell lines ( c ) and in HGSOC ( d ). qRT–PCR data are shown as normalized cycle threshold centred to the mean (ΔΔCt). Spearman correlation coefficients ρ (rho) and corresponding P- values are indicated on each graph. n =3 independent experiments per cell line, except for OVCAR3 cells, n =2. ( e , f ) Effect of the transcription inhibitor actinomycin D (Act D) on the levels of miR-141 (grey) or miR-200c (black) ( e ) and their corresponding primary transcript, pri-miR-200c-141 ( f ), under untreated conditions (NT) or following 3 h of H 2 O 2 treatment (+H 2 O 2 ). Cells were pretreated for 4 h with Act D or dimethylsulphoxide (control). qRT–PCR data are shown as fold change±s.d. of treated compared with untreated cells. n≥ 2 independent experiments per cell line. Full size image miR-200c/141 transcription is coupled to PTPN6 expression We first observed that neither ZEB nor TP53 protein was involved in the upregulation of miR-200c/141 by oxidative stress in ovarian cancer cell lines ( Supplementary Fig. 1c ), suggesting that the mechanism involved was complementary to those previously described. We thus analysed the genomic locus from which these miRNAs are transcribed ( Fig. 2a ). We first tested whether transcription of the miR-200c/141 neighbouring genes could be affected by acute oxidative stress. We observed that the transcription of the immediate upstream gene, PTPN6 , was significantly increased following H 2 O 2 treatment, whereas the downstream gene, PHB2 , remained invariant ( Fig. 2b ). Interestingly, the kinetics of PTPN6 upregulation was strikingly similar to this one of the miR-200c/141 primary transcript, pri-miR-200c-141 ( Fig. 2b ). The coupling between PTPN6 and miR-200c/141 primary transcripts upon stress was observed in 12 different cell lines ( Fig. 2b and Supplementary Fig. 1b ), suggesting a conserved mechanism of co-regulation in mammals. Moreover, this coupled transcription was also observed upon treatments increasing reactive oxygen species ( Fig. 2c ). Furthermore, the remarkable association between pri-miR-200c-141 and pri-PTPN6 transcription was not restricted to stress conditions but also observed at basal state in ovarian and breast cancer cell lines ( Fig. 2d ). We further confirmed this result by validating the correlation between PTPN6 and miR-200c/141 levels in publicly available data sets from two large cell line panels, the NCI60 panel and the Sanger Cell Line Project ( Fig. 2e,f ). Taken together, these results demonstrate that miR-200c/141 and PTPN6 transcriptions are tightly associated in a variety of cell lines at basal state and upon oxidative stress. Figure 2: pri-miR-200c-141 expression correlates with PTPN6 transcription. ( a ) Schematic representation (adapted from http://genome.ucsc.edu ) of miR-200c/141 genomic locus showing upstream ( PTPN6 ) and downstream ( PHB2, SCARNA12 ) neighbouring genes in human and mouse species, as indicated. Genomic positions, scale and genome versions used ( hg19 and mm10 ) are indicated on the top. Horizontal arrows indicate the sense of transcription. Coding exons are indicated as blocks connected by horizontal lines representing introns, and arrowheads showing sense of transcription. Untranslated regions are presented by thinner blocks. P1 and P2 indicate the alternative promoters used for PTPN6 transcription in non-haematopoietic and haematopoietic cells, respectively. ( b ) Kinetics of accumulation of pri-miR-200c-141, pri-PTPN6 and pri-PHB2 primary transcripts following H 2 O 2 treatment in human ovarian cancer cells (SKOV3, OVCA433), human (WI38, MRC5) and mouse fibroblasts. qRT–PCR data are means of fold changes (normalized to untreated and expressed as log 2 )±s.e.m. n =3 independent experiments at least, except for OVCA433, n =2 (in this case error bars indicate range of data). Sequences of the primers from mouse or human origins (pri-miR-200c-141F/R and pri-PTPN6/Ptpn6(2) F/R) used are given in Supplementary Table 2 . ( c ) Effect of different stresses on pri-miR-200c-141, pri-Ptpn6 and pri-Phb2 primary transcript levels. MSB, menadione sodium bisulfite. qRT–PCR data are shown as fold change±s.d. following treatments, compared with untreated fibroblasts (NT). n =3 independent experiments. ( d ) Scatter plot showing correlation between pri-PTPN6 and pri-miR-200c-141 primary transcript levels in ovarian and breast cancer cells. qRT–PCR data are shown as normalized cycle threshold centred to the mean (ΔΔCt). ( e , f ) Scatter plots showing that miR-200c (left) and miR-141 (right) levels are correlated with PTPN6 mRNA levels in NCI-60 panel of cell lines ( e ) and Sanger Cell Line Project ( f ). Spearman correlation coefficients ρ (rho) and P- values are indicated on each graph. Full size image Pri-miR-200/PTPN6 transcripts are coupled in ovarian cancer As miR-200c/141 have been repeatedly defined as key regulators of human ovarian tumorigenesis [5] , [7] , [9] , [10] , [15] , [32] , [33] , [34] , [35] , [36] , we next wondered whether the correlation of expression between miR-200c/141 and PTPN6 was also observed in HGSOC. We first observed that the expression of the two miRNAs ( Fig. 3a ) and their corresponding primary transcript ( Fig. 3b ) were correlated with PTPN6 mRNA levels in a cohort of 107 HGSOC ( Fig. 3a,b ). Correlation between miR-200c/141 and PTPN6 expression was further validated in the publicly available The Cancer Genome Atlas (TCGA) database [51] composed by 574 HGSOC patients ( Fig. 3c and details of the cohort are given in Supplementary Table 1 ). 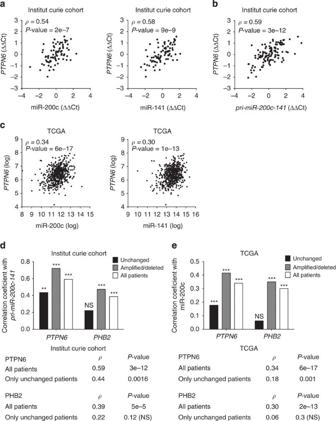Figure 3:miR-200c/141expression correlates withPTPN6in HGSOC, independently of genomic alterations. (a) Scatter plots showing thatPTPN6mRNA levels are correlated with miR-200c (left) and miR-141 (right) levels in ovarian tumours (Institut Curie cohort). qRT–PCR data are shown as normalized cycle threshold centred to the mean (ΔΔCt). (b) Scatter plot showing correlation between levels ofPTPN6andpri-miR-200c-141primary transcripts in ovarian tumours (Institut Curie cohort). qRT–PCR data are shown as normalized cycle threshold centred to the mean (ΔΔCt). Sequences of the primers (pri-miR-200c-141F/Randpri-PTPN6(1) F/R) used for detection of primary transcripts are given inSupplementary Table 2. (c) Scatter plots showing thatPTPN6mRNA levels are correlated with miR-200c (left) and miR-141 (right) levels in ovarian tumours of the TCGA cohort. Microarray data were obtained from the TCGA portal.pri-miR-200c-141levels were not available. (d,e) Correlation coefficients betweenPTPN6orPHB2mRNA levels withpri-miR-200c-141primary transcript levels in ovarian tumours from the Institut Curie (d) and TCGA (e) cohorts. Correlations take into account either all patients (white) or patient subgroups defined according to their genomic status: amplified/deleted (grey), patients with amplifications or deletions in the region of interest; unchanged (black), patients with no genomic alteration in the region of interest. Numbers below indicate Spearman correlation coefficientsρ(rho) and correspondingP-values per gene (PTPN6orPHB2) for each subgroup of patients in each cohort. NS, not significant. Figure 3: miR-200c/141 expression correlates with PTPN6 in HGSOC, independently of genomic alterations. ( a ) Scatter plots showing that PTPN6 mRNA levels are correlated with miR-200c (left) and miR-141 (right) levels in ovarian tumours (Institut Curie cohort). qRT–PCR data are shown as normalized cycle threshold centred to the mean (ΔΔCt). ( b ) Scatter plot showing correlation between levels of PTPN6 and pri-miR-200c-141 primary transcripts in ovarian tumours (Institut Curie cohort). qRT–PCR data are shown as normalized cycle threshold centred to the mean (ΔΔCt). Sequences of the primers ( pri-miR-200c-141F/R and pri-PTPN6(1) F/R ) used for detection of primary transcripts are given in Supplementary Table 2 . ( c ) Scatter plots showing that PTPN6 mRNA levels are correlated with miR-200c (left) and miR-141 (right) levels in ovarian tumours of the TCGA cohort. Microarray data were obtained from the TCGA portal. pri-miR-200c-141 levels were not available. ( d , e ) Correlation coefficients between PTPN6 or PHB2 mRNA levels with pri-miR-200c-141 primary transcript levels in ovarian tumours from the Institut Curie ( d ) and TCGA ( e ) cohorts. Correlations take into account either all patients (white) or patient subgroups defined according to their genomic status: amplified/deleted (grey), patients with amplifications or deletions in the region of interest; unchanged (black), patients with no genomic alteration in the region of interest. Numbers below indicate Spearman correlation coefficients ρ (rho) and corresponding P- values per gene ( PTPN6 or PHB2 ) for each subgroup of patients in each cohort. NS, not significant. Full size image Genomic amplifications have been previously described in HGSOC on the chromosome 12p13, including the genomic locus from which the miR-200c/141 and PTPN6 are transcribed [51] . We hypothesized that genomic amplification could contribute to the observed correlation between PTPN6 and pri-miR-200c-141 transcription levels in these tumours. We thus computed the Transcription Correlation Scores (TCS) of this genomic region ( Supplementary Fig. 2 ), TCS reflecting the degree of correlation of each gene with its neighbours, as defined previously [52] . We observed a peak of correlation in the TCS map around the PTPN6 gene in both Institut Curie and TCGA cohorts ( Supplementary Fig. 2a,b ). We analysed the copy number alterations of HGSOC samples and classified the patients, referred to as unchanged or amplified/deleted, according to their genomic status in this specific region ( Supplementary Fig. 2e ). When we restricted the analysis to patients of the unchanged subgroup, the TCS peak observed around the PTPN6 gene with all patients was lost in both cohorts ( Supplementary Fig. 2c,d ), revealing this peak was indeed because of genomic alterations. In contrast, the correlation between PTPN6 and pri-miR-200c-141 transcription was maintained in patients with no copy number alteration in this locus (unchanged subgroup; Fig. 3d ). Interestingly, in this subgroup, the correlation was restricted to PTPN6 , and was not observed with PHB2 , the downstream gene ( Fig. 3d ). Accordingly, the same findings were obtained from the TCGA cohort ( Fig. 3e ), strengthening the validity of such data. In this cohort, mature miRNA levels were analysed, as pri-miRNA-200c-141 levels were not available. It is noteworthy that PTPN6 was ranked the 13th-most correlated gene with miR-200c among the 12,044 genes tested, in the TCGA cohort. Together, these results indicate that the transcriptional co-regulation between PTPN6 and miR-200c/141 is a relevant process for the expression of the two miRNAs in HGSOC independently of genomic alterations. Two complementary mechanisms drive miR-200c/141 expression To explain the tight correlation between pri-miR-200c-141 and PTPN6 primary transcripts, we considered two non-exclusive hypotheses ( Supplementary Fig. 2f ). In the first hypothesis, the PTPN6 primary transcription bypasses its usual polyadenylation site, thereby promoting the downstream expression of miR-200c/141. In this case, miR-200c/141 transcription results from either an APA of PTPN6 mRNA or a late termination of PTPN6 transcription. In the second hypothesis, pri-PTPN6 and pri-miR-200c-141 primary transcripts are produced from two independent but co-regulated promoters. This co-regulation could be mediated by a spatial DNA conformation, favouring shared regulation by common transcription factors and/or epigenetic marks. The two mechanisms could work together, with PTPN6 bypass favouring the transcription initiation at the miRNA locus, for example. It is worth noting that the PTPN6 gene has two alternative promoters ( Fig. 2a ). Here, we were interested in the most 5′ one, also called P1, which is the one used in almost all cell types, except haematopoietic cells, in which P2 is active [53] . We will refer below to PTPN6 P1 promoter as PTPN6 promoter. The polyadenylation site of the PTPN6 gene is bypassed We first demonstrated the existence of a transcript, downstream of the polyadenylation site of the PTPN6 gene and upstream of the miR-200c/141-coding region (schema Fig. 4a ). This intermediate transcript (assessed with Set 1 primers, compatible with quantitative reverse transcription–PCR (qRT–PCR) experiments) accumulated with the same kinetics as PTPN6 primary transcript upon oxidative stress ( Fig. 4b , left panel, and Supplementary Fig. 3a,b , left panel). As expected according to the clear correlation between PTPN6 and pri-miR-200c-141 , this intermediate transcript followed also the same kinetics as pri-miR-200c-141 ( Fig. 4b , right panel, and Supplementary Fig. 3b , right panel). We thus speculated that this intermediate transcript was the result of a transcriptional read-through from the PTPN6 gene. In agreement with the assumption that PTPN6 read-through led to the transcription of the downstream miR-200c/141, this intermediate transcript was also correlated with the pri-miR-200c-141 in HGSOC ( Fig. 4c , right). Moreover, we also detected a significant correlation between the expression levels of this intermediate transcript and PTPN6 primary transcript in HGSOC ( Fig. 4c , left). Importantly, a read-through from the PTPN6 gene was also detected in RNA-seq data generated from a set of cell lines in the ENCODE project and visualized using the UCSC Genome Browser ( Supplementary Fig. 4 ). The levels of expression of the intermediate transcript, while being much lower than mature (exonic) PTPN6 mRNA as expected, reached the same expression rate as the pri-PTPN6 primary (intronic) transcript ( Supplementary Fig. 4 ). We next demonstrated that this intermediate transcript resulted from the bypass of the usual polyadenylation site of the PTPN6 gene ( Fig. 4d,e ). Indeed, we detected both spliced and unspliced transcripts extending from PTPN6 -coding sequence to the downstream region of its usual polyadenylation site, in both mouse and human cells at basal states and following H 2 O 2 exposure ( Set 2 primers, Fig. 4d and Supplementary Fig. 3c ). Importantly, the same type of transcript was also detected in human HGSOC ( Fig. 4d , bottom). Furthermore, we confirmed that these bypassed PTPN6 transcripts reached the pri-miR-200c-141 sequence both in cell lines and in HGSOC ( Set 3 primers, Fig. 4e and Supplementary Fig. 3d ), thus showing that PTPN6 read-through could indeed reach the miR-200c/141 locus and impact directly pri-miR-200c-141 expression. The products amplified using the Set 2 and Set 3 couples of primers were cloned and sequenced, in order to verify that they corresponded to the region located between PTPN6 3′-end and miR-200c-141 5′-end. It was noteworthy that this intermediate transcript was detected at the same levels by quantitative PCR (qPCR) by using either random hexamers or oligo dT in the reverse transcription reaction, suggesting it was polyadenylated. Consistently, using the 3′ Rapid Amplification of cDNA Ends (RACE) methodology, we identified APA sites reached by the pri-PTPN6/pri-miR-200c-141 transcript ( Supplementary Fig. 5a,b ). These observations thus demonstrate that the read-through transcription from the PTPN6 gene can reach the miR-200c-141 encoding unit and that the levels of these transcripts are comparable. According to these results, the transcriptional co-regulation between PTPN6 and miR-200c-141 genes can result from late termination of transcription by RNA-polymerase II or APA (hypothesis 1, Supplementary Fig. 2f ). 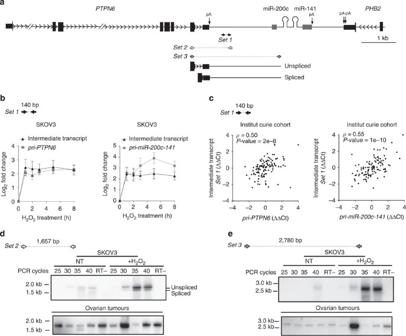Figure 4: The usual polyadenylation site of thePTPN6gene is bypassed. (a) Schematic representation (adapted from UCSC browser:https://genome.ucsc.edu) of the human genomic locus showingmiR-200c/141and their neighbouring genes,PTPN6andPHB2. Black and grey boxes represent exons and ESTs, respectively. Polyadenylation sites (pA) are indicated (see details inSupplementary Fig. 5).Set 1,Set 2andSet 3primers allow detection of the Intermediate transcript by qPCR (Set 1) and by PCR (Set 2,Set 3), respectively. Sequences are given inSupplementary Table 2. Lengths of the amplified products usingSet 1–3primers are indicated in base pairs (bp) inb,d,e. (b) Kinetics of accumulation of the intermediate transcript detected usingSet 1primers upon H2O2treatment in SKOV3 ovarian cancer cells and compared withpri-PTPN6(left) orpri-miR-200c/141(right) primary transcripts. qRT–PCR data are means of fold changes (normalized to untreated and expressed as log2)±s.e.m.n≥3 independent experiments. (c) Correlation plot showing that RNA levels of the intermediate transcript are correlated withpri-PTPN6(left) andpri-miR-200c-141(right) primary transcript levels in ovarian tumours (Institut Curie cohort). (d,e) PCR reactions usingSet 2(d) andSet 3(e) primers showing intermediate transcripts spanning fromPTPN63′-end and reaching miR-200c/141 locus. Representative amplifications using cDNA from untreated (NT) or H2O2-treated (+H2O2) SKOV3 cells (up) and ovarian tumours (bottom). Numbers of PCR cycles performed are indicated on the top. RT- indicates control without the reverse transcriptase enzyme. The amplified fragments have been cloned and sequenced to verify that they correspond to the intermediate transcript. Figure 4: The usual polyadenylation site of the PTPN6 gene is bypassed. ( a ) Schematic representation (adapted from UCSC browser: https://genome.ucsc.edu ) of the human genomic locus showing miR-200c/141 and their neighbouring genes, PTPN6 and PHB2 . Black and grey boxes represent exons and ESTs, respectively. Polyadenylation sites (pA) are indicated (see details in Supplementary Fig. 5 ). Set 1 , Set 2 and Set 3 primers allow detection of the Intermediate transcript by qPCR ( Set 1 ) and by PCR ( Set 2 , Set 3) , respectively. Sequences are given in Supplementary Table 2 . Lengths of the amplified products using Set 1–3 primers are indicated in base pairs (bp) in b , d , e . ( b ) Kinetics of accumulation of the intermediate transcript detected using Set 1 primers upon H 2 O 2 treatment in SKOV3 ovarian cancer cells and compared with pri-PTPN6 (left) or pri-miR-200c/141 (right) primary transcripts. qRT–PCR data are means of fold changes (normalized to untreated and expressed as log 2 )±s.e.m. n ≥3 independent experiments. ( c ) Correlation plot showing that RNA levels of the intermediate transcript are correlated with pri-PTPN6 (left) and pri-miR-200c-141 (right) primary transcript levels in ovarian tumours (Institut Curie cohort). ( d , e ) PCR reactions using Set 2 ( d ) and Set 3 ( e ) primers showing intermediate transcripts spanning from PTPN6 3′-end and reaching miR-200c/141 locus. Representative amplifications using cDNA from untreated (NT) or H 2 O 2 -treated (+H 2 O 2 ) SKOV3 cells (up) and ovarian tumours (bottom). Numbers of PCR cycles performed are indicated on the top. RT- indicates control without the reverse transcriptase enzyme. The amplified fragments have been cloned and sequenced to verify that they correspond to the intermediate transcript. Full size image PTPN6 read-through drives pri-miR-200c-141 transcription We next wondered in which proportion the read-through from the PTPN6 gene participates to miR-200c/141 transcription. We quantified the expression rates of each RNA entity detected along PTPN6 and miR-200c-141 genomic locus, namely the pri-PTPN6 primary transcript, the intermediate transcript (RNA detected downstream PTPN6 polyadenylation signal and upstream miR-200c/141 promoter) and the pri-miR-200c-141 primary transcript, whose synthesis could result from both PTPN6 read-through and transcription from miR-specific promoter ( Fig. 5a ). Two experimental proceedings were adopted to quantify these weakly expressed molecules. First, nuclear RNA was used, in order to increase sensitivity of the assay. Second, pri-miR-200c-141 amount was evaluated using qPCR primers located outside of a previously described expressed sequence tag (EST) (grey boxes Fig. 5a ). This avoided bias related to different RNA stability (when comparing EST and intronic RNA) and allowed comparison with intronic pri-PTPN6 and intermediate transcript in absolute quantities. Based on standard curves obtained on serial dilutions of a bacterial artificial chromosome (BAC) DNA corresponding to the same genomic locus ( Supplementary Fig. 6a ), we first observed that the quantity of the intermediate transcript was equivalent to the level of the pri-PTPN6 and pri-miR-200c-141 primary transcripts in SKOV3 ovarian cancer cells at basal state ( Fig. 5b ). Indeed, in these cells, although the expression rate was faint, data indicated that all molecules of pri-PTPN6 primary transcript were able to bypass PTPN6 polyadenylation signal (ratio Intermediate transcript/pri-PTPN6 =1; Fig. 5c ). Moreover, all intermediate transcripts gave rise to pri-miR-200c-141 primary transcripts (ratio pri-miR-200c-141/Intermediate transcript =1; Fig. 5c; see also Fig. 9a for schematic representation of the data). Upon H 2 O 2 exposure, PTPN6 transcription initiation (evaluated by the pri-PTPN6 transcript quantity) increased fivefold ( Fig. 5d ), whereas the levels of the intermediate transcript was only induced threefold ( Figs 5d,e ). Indeed, only 56% of PTPN6 primary transcripts were able to bypass PTPN6 polyadenylation signal, suggesting that PTPN6 read-through was reduced by oxidative stress. Still, the totality of the 56% intermediate transcript contributed to pri-miR-200c-141 primary transcription (ratio pri-miR-200c-141/Intermediate transcript =1) in SKOV3 following oxidative stress ( Fig. 5e ). 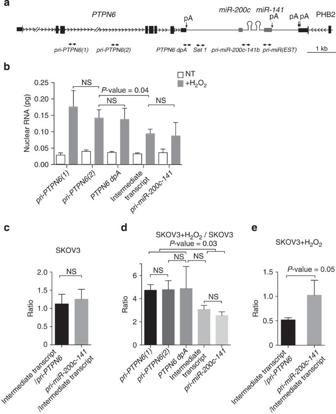Figure 5: Quantification of primary transcripts detected alongPTPN6andmiR-200c/141genomic locus. (a) Schematic representation of the humanPTPN6-miR-200c/141genomic locus, as shown and explained inFig. 4a. (b) Quantities of primary transcripts detected alongPTPN6andmiR-200c-141genomic locus, assessed by qPCR using cDNA from nuclear RNA of untreated (NT) or H2O2-treated SKOV3 cells.pri-PTPN6(1)andpri-PTPN6(2)primers detect thepri-PTPN6primary transcript,PTPN6 dpAoverlapsPTPN6polyadenylation signal,Set 1allows detection of the Intermediate transcript andpri-miR-200c-141bdetects thepri-miR-200c-141primary transcript. Quantifications were assessed using standard curves shown inSupplementary Fig. 6. Quantities are expressed in picogram (pg). Data are means of±s.e.m.n=6 independent experiments per cell line.P-values are from Student’st-test. (c,e) Ratios of quantities of intermediate transcript versuspri-PTPN6primary transcript andpri-miR-200c-141/Intermediate transcript, as indicated in SKOV3 cells (c) and SKOV3+H2O2(e). (d) Ratios of quantities of each primary transcript (as indicated) in SKOV3+H2O2versus SKOV3 cells.P-values are from Student’st-test. Data are meansn=6 independent experiments. NS, not significant. Figure 5: Quantification of primary transcripts detected along PTPN6 and miR-200c/141 genomic locus. ( a ) Schematic representation of the human PTPN6-miR-200c/141 genomic locus, as shown and explained in Fig. 4a . ( b ) Quantities of primary transcripts detected along PTPN6 and miR-200c-141 genomic locus, assessed by qPCR using cDNA from nuclear RNA of untreated (NT) or H 2 O 2 -treated SKOV3 cells. pri-PTPN6(1) and pri-PTPN6(2) primers detect the pri-PTPN6 primary transcript, PTPN6 dpA overlaps PTPN6 polyadenylation signal, Set 1 allows detection of the Intermediate transcript and pri-miR-200c-141b detects the pri-miR-200c-141 primary transcript. Quantifications were assessed using standard curves shown in Supplementary Fig. 6 . Quantities are expressed in picogram (pg). Data are means of±s.e.m. n =6 independent experiments per cell line. P -values are from Student’s t -test. ( c , e ) Ratios of quantities of intermediate transcript versus pri-PTPN6 primary transcript and pri-miR-200c-141 /Intermediate transcript, as indicated in SKOV3 cells ( c ) and SKOV3+H 2 O 2 ( e ). ( d ) Ratios of quantities of each primary transcript (as indicated) in SKOV3+H 2 O 2 versus SKOV3 cells. P -values are from Student’s t -test. Data are means n =6 independent experiments. NS, not significant. Full size image Figure 9: Model: miR-200c and miR-141 are co-transcribed with PTPN6 by two complementary mechanisms, intergenic DNA-looping and transcriptional read-through. ( a ) Schematic representation of the PTPN6 - miR-200c/141 genomic locus and results obtained by quantitative analyses of the different primary transcripts detected along the locus, including pri-PTPN6 primary transcript, Intermediate transcript, pri-miR-200c-141 primary transcript and pri-miR(EST) exonic isoform, corresponding to previously described ESTs . Double arrows represent the primers used for detection of the transcripts. 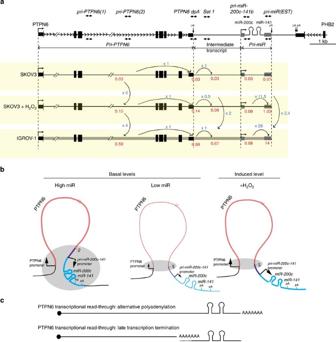Figure 9: Model: miR-200c and miR-141 are co-transcribed withPTPN6by two complementary mechanisms, intergenic DNA-looping and transcriptional read-through. (a) Schematic representation of thePTPN6-miR-200c/141genomic locus and results obtained by quantitative analyses of the different primary transcripts detected along the locus, includingpri-PTPN6primary transcript, Intermediate transcript,pri-miR-200c-141primary transcript and pri-miR(EST) exonic isoform, corresponding to previously describedESTs. Double arrows represent the primers used for detection of the transcripts. Quantities (in picograms) of each RNA entity detected alongPTPN6andmiR-200c-141genomic locus are shown in red. Fold changes are expressed in blue. (b) The short-range intergenic DNA-looping formed by the physical interaction betweenPTPN6andmiR-200c/141promoters is associated with the transcription rate of the two genes. The grey-shaded ovals indicate the genomic regions, which have been defined as interacting with each other, according to 3C experiments. In cells characterized by high basal levels ofPTPN6andmiR-200c/141transcription, thePTPN6promoter can interact with a large region including the 3′-end of thePTPN6gene, themiR-200c/141promoter and downstream sequences. In cells expressing low basal levels of the two genes, the interaction is restricted to the 3′-end ofPTPN6and does not includemiR-200c/141. This conformation is not altered by the increased transcription upon oxidative stress (+H2O2), suggesting the existence of another mechanism is responsible for the co-expression ofmiR-200c/141andPTPN6following oxidative stress. (c) The transcriptional co-regulation betweenPTPN6andmiR-200c/141can also be mediated by a transcriptional read-through of thePTPN6gene. This is highlighted by the intermediate transcripts, linkingPTPN6tomiR-200c/141, we identified. These intermediate transcripts can result from alternative polyadenylation or late termination of transcription by RNA-polymerase II, as schematically represented. Quantities (in picograms) of each RNA entity detected along PTPN6 and miR-200c-141 genomic locus are shown in red. Fold changes are expressed in blue. ( b ) The short-range intergenic DNA-looping formed by the physical interaction between PTPN6 and miR-200c/141 promoters is associated with the transcription rate of the two genes. The grey-shaded ovals indicate the genomic regions, which have been defined as interacting with each other, according to 3C experiments. In cells characterized by high basal levels of PTPN6 and miR-200c/141 transcription, the PTPN6 promoter can interact with a large region including the 3′-end of the PTPN6 gene, the miR-200c/141 promoter and downstream sequences. In cells expressing low basal levels of the two genes, the interaction is restricted to the 3′-end of PTPN6 and does not include miR-200c/141 . This conformation is not altered by the increased transcription upon oxidative stress (+H 2 O 2 ), suggesting the existence of another mechanism is responsible for the co-expression of miR-200c/141 and PTPN6 following oxidative stress. ( c ) The transcriptional co-regulation between PTPN6 and miR-200c/141 can also be mediated by a transcriptional read-through of the PTPN6 gene. This is highlighted by the intermediate transcripts, linking PTPN6 to miR-200c/141 , we identified. These intermediate transcripts can result from alternative polyadenylation or late termination of transcription by RNA-polymerase II, as schematically represented. Full size image Finally, we evaluated the role of PTPN6 transcription and read-through in stress-induced pri-miR-200c-141 transcription by using the CRISPR/Cas9 technology ( Fig. 6 ). In that aim, we deleted the genomic region containing the two promoters (P1 and P2) driving PTPN6 transcription in epithelial and haematopoietic cells, respectively ( Fig. 6a ). We decided to avoid the use of a selection gene, which would have required the insertion of an independent promoter with the risk of an ectopic transcriptional start in the PTPN6 locus. We selected two stable cell lines from parental SKOV3 cells (SKOV3-Δ1 and SKOV3-Δ2) based on PCR and qPCR genotyping ( Fig. 6b–d ). Genomic deletion of PTPN6 promoters reduced significantly PTPN6 upregulation by oxidative stress ( Fig. 6e , left), as expected for a transcriptional-dependent regulation. Importantly, depletion of PTPN6 promoters also prevented the induction of both the intermediate transcript and the pri-miR-200c-141 transcript ( Fig. 6e , middle and right). These experiments demonstrate that PTPN6 transcription is required for pri-miR-200c-141 upregulation upon stress. 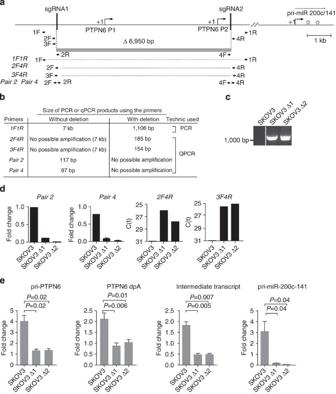Taken as a whole, these results show that the transcriptional read-through from the PTPN6 gene leads to the transcription of the pri-miR-200c-141 and explains, at least in part, how PTPN6 transcription could regulate miR-200c/141 levels following oxidative stress in ovarian cancer cells. Figure 6:PTPN6transcription is necessary forpri-miR-200c-141transcription. (a) Schematic representation of the genomic deletion of 6,950 bp (grey box) targeting thePTPN6promoter region using the CRISPR/Cas9 technology. Are represented the P1 and P2 promoters, expressed in epithelial and haematopoietic cells, respectively, as well as the position of the target-specific CRISPR guide RNAs (sgRNA). Double arrows represent the position and orientation of the primers used. (b) Table summarizing the sizes of the PCR- and qPCR-amplification products used for genotyping. (c,d) Characterization of 2 SKOV3-derived cell lines (SKOV3-Δ1, SKOV3-Δ2) among 63 individual clones tested after depletion ofPTPN6promoter genomic region using the CRISPR/Cas9 technology. (c) Fragment of 1,106 pb amplified by PCR from genomic DNA of SKOV3-Δ1 and SKOV3-Δ2 cell lines using1F1Rprimers. As expected, no amplification was seen in parental SKOV3 cells. (d) qPCR-based genotyping results from genomic DNA of SKOV3, SKOV3-Δ1 and SKOV3-Δ2 cell lines. Amplified products obtained from primers described inb.Pair 2andPair 4primers are specific of the deleted genomic region; fragments from 2F4R and 3F4R primers can be amplified only in case of deletion. qPCR data are shown as fold change normalized to SKOV3 forPair2andPair4primers and as normalized cycle threshold for2F4Rand3F4Rprimers, as the signal is null in SKOV3 parental cells. (e) qRT–PCR data showingpri-PTPN6,PTPN6 dpA,intermediate transcriptandpri-miR-200c-141primary transcripts. Data are from SKOV3, SKOV3-Δ1 and SKOV3-Δ2 cell lines, following 3 h of H2O2treatment. Data are means of fold changes (normalized to untreated and expressed as log2)±s.e.m.n=3 independent experiments per cell line.P-values are from Student’st-test. Figure 6: PTPN6 transcription is necessary for pri-miR-200c-141 transcription. ( a ) Schematic representation of the genomic deletion of 6,950 bp (grey box) targeting the PTPN6 promoter region using the CRISPR/Cas9 technology. Are represented the P1 and P2 promoters, expressed in epithelial and haematopoietic cells, respectively, as well as the position of the target-specific CRISPR guide RNAs (sgRNA). Double arrows represent the position and orientation of the primers used. ( b ) Table summarizing the sizes of the PCR- and qPCR-amplification products used for genotyping. ( c , d ) Characterization of 2 SKOV3-derived cell lines (SKOV3-Δ1, SKOV3-Δ2) among 63 individual clones tested after depletion of PTPN6 promoter genomic region using the CRISPR/Cas9 technology. ( c ) Fragment of 1,106 pb amplified by PCR from genomic DNA of SKOV3-Δ1 and SKOV3-Δ2 cell lines using 1F1R primers. As expected, no amplification was seen in parental SKOV3 cells. ( d ) qPCR-based genotyping results from genomic DNA of SKOV3, SKOV3-Δ1 and SKOV3-Δ2 cell lines. Amplified products obtained from primers described in b . Pair 2 and Pair 4 primers are specific of the deleted genomic region; fragments from 2F4R and 3F4R primers can be amplified only in case of deletion. qPCR data are shown as fold change normalized to SKOV3 for Pair2 and Pair4 primers and as normalized cycle threshold for 2F4R and 3F4R primers, as the signal is null in SKOV3 parental cells. ( e ) qRT–PCR data showing pri-PTPN6 , PTPN6 dpA , intermediate transcript and pri-miR-200c-141 primary transcripts. Data are from SKOV3, SKOV3-Δ1 and SKOV3-Δ2 cell lines, following 3 h of H 2 O 2 treatment. Data are means of fold changes (normalized to untreated and expressed as log 2 )±s.e.m. n =3 independent experiments per cell line. P -values are from Student’s t -test. Full size image PTPN6 and miR-200c/141 promoters share epigenetic marks As described above, we observed a strict correlation between PTPN6 and pri-miRNA-200c-141 transcription. It has been previously shown that miR-200c/141 transcription can be initiated downstream from the PTPN6 gene and regulated by an independent promoter [11] , [15] , [37] , [38] , [39] . In addition to the read-through of the PTPN6 gene, we thus next checked whether the transcription of pri-miR-200c-141 could be initiated at its closest transcriptional start site (TSS). Indeed, PTPN6 bypass could reach miR-200c/141 locus but also favour transcription initiation of poised RNA Polymerase II on miRNA TSS. Using 5′RACE method, we were able to confirm the existence of a capped mRNA entity, whose 5′-extremity was compatible with previously identified EST located upstream of miR-200c ( Supplementary Fig. 5a ). Consistently, chromatin immunoprecipitation (ChIP) experiments confirmed RNA polymerase II recruitment at PTPN6 P1 and miR 200c/141 promoters ( Supplementary Fig. 5c,d ). Thus, in addition to transcripts generated through the bypass of the PTPN6 polyA site, miR-200c/141 expression can also be initiated at their independent promoter. As we observed a striking correlation between PTPN6 and pri-miR-200c-141 transcription, we next wondered if the two promoters could share regulatory mechanisms. By performing methylated-DNA immunoprecipitation (MeDIP) experiments, we showed that PTPN6 - and miR-200c/141 -specific promoters were both methylated in cell lines with low expression of miR-200c/141 and demethylated in cells characterized by high-miR-200c/141 expression ( Fig. 7a,b ), confirming previous results [40] , [42] , [43] . Accordingly, both PTPN6 and pri-miRNA-200c-141 genes were upregulated upon treatment with a DNA demethylating agent, 5-aza-2'-deoxycytidine ( Supplementary Fig. 7a ). As expected, the PTPN6 haematopoietic promoter P2 is highly methylated in ovarian cancer cells. Moreover, the active histone methylation marks H3K9Ac and H3K4me3 enrichment were in complete agreement with DNA methylation status in all cell lines tested ( Fig. 7c,d ). Together, these results indicate that the PTPN6 and miR-200c/141 promoters could be under equivalent epigenetic regulation. We further extended this observation to 46 non-haematopoietic cell lines of the ENCODE project, in which the methylation states of PTPN6 and miR-200c/141 promoters were correlated ( Supplementary Fig. 7b ). Finally, in HGSOC from the TCGA cohort, although miR-200c/141 expression levels were globally high, the methylation status of the PTPN6 promoter was significantly negatively correlated with the miR-200c/141 expression levels ( Supplementary Fig. 7c ), highlighting the relevance of our findings not only in cultured cell lines but also in human cancers. 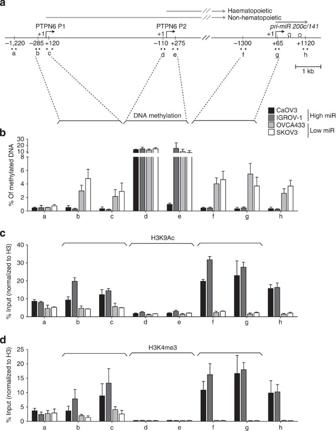In conclusion, PTPN6 and miR-200c/141 regulatory regions exhibit similar epigenetic marks and might share epigenetic-regulatory mechanisms. Figure 7: The same epigenetic marks are associated withPTPN6andmiR-200c/141promoters. (a) Schematic representation ofPTPN6andpri-miR-200c-141genomic organization showing the localization of the primers (referred to as a–h) used for MeDIP and ChIP experiments. Broken arrows representmiR-200c/141andPTPN6promoters, PTPN6-P1 and PTPN6-P2 being active in non-haematopoietic and haematopoietic cells, respectively. +1 indicate the start sites ofPTPN6andmiR-200c/141transcription. Positions of the primers relative to each start site are indicated. Sequences of the primers are listed inSupplementary Table 2. (b) Percentage of methylated DNA, defined by MeDIP experiments using primers indicated inain ovarian cancer cell lines characterized by high (CaOV3, IGROV-1) or low (OVCA433, SKOV3) expression ofPTPN6andmiR-200c/141, as indicated. Values are means±s.e.m.n=6 independent experiments per cell line, except for CaOV3,n=2 (in this case error bars indicate range of data). (c,d) ChIP experiment using anti-H3K9Ac- (c) and H3K4me3-specific antibodies (d) in ovarian cancer cell lines, as indicated. Values are presented as percentage (%) of input DNA (amount of DNA extracted per experiment), normalized to DNA amount immunoprecipitated using anti-histone H3 antibody. Values are means±s.e.m.n=3 independent experiments at least per cell line, except for CaOV3,n=2 (in this case error bars indicate range of data). Figure 7: The same epigenetic marks are associated with PTPN6 and miR-200c/141 promoters. ( a ) Schematic representation of PTPN6 and pri-miR-200c-141 genomic organization showing the localization of the primers (referred to as a–h) used for MeDIP and ChIP experiments. Broken arrows represent miR-200c/141 and PTPN6 promoters, PTPN6-P1 and PTPN6-P2 being active in non-haematopoietic and haematopoietic cells, respectively. +1 indicate the start sites of PTPN6 and miR-200c/141 transcription. Positions of the primers relative to each start site are indicated. Sequences of the primers are listed in Supplementary Table 2 . ( b ) Percentage of methylated DNA, defined by MeDIP experiments using primers indicated in a in ovarian cancer cell lines characterized by high (CaOV3, IGROV-1) or low (OVCA433, SKOV3) expression of PTPN6 and miR-200c/141 , as indicated. Values are means±s.e.m. n =6 independent experiments per cell line, except for CaOV3, n =2 (in this case error bars indicate range of data). ( c , d ) ChIP experiment using anti-H3K9Ac- ( c ) and H3K4me3-specific antibodies ( d ) in ovarian cancer cell lines, as indicated. Values are presented as percentage (%) of input DNA (amount of DNA extracted per experiment), normalized to DNA amount immunoprecipitated using anti-histone H3 antibody. Values are means±s.e.m. n =3 independent experiments at least per cell line, except for CaOV3, n =2 (in this case error bars indicate range of data). Full size image PTPN6 and miR-200c/141 promoters interact via a DNA loop We finally wondered how their promoters of the PTPN6 and miR-200c/141 genes could be so finely co-regulated. We hypothesized that co-transcription of the two genes could result from a physical interaction between their promoters, thus facilitating regulation by common molecules, such as epigenetic regulators. To test this hypothesis, we performed chromosome conformation capture (3C) experiments ( Fig. 8 ) that quantifies interaction frequency between genomic regions with high sensitivity for short-range chromatin interaction [54] . We first performed 3C experiments on the IGROV-1 ovarian cancer cell line expressing high levels of PTPN6 and miR-200c/141 transcripts ( Fig. 8c,d ; see Supplementary Fig. 1d and Supplementary Fig. 6c for comparative quantification of PTPN6 and miR-200c-141 primary transcripts in IGROV-1 and SKOV3 cell lines). Interestingly, we uncovered an interaction between PTPN6 - and miR-200c/141 -specific promoters, using a primer anchor (anchor 1) located at the miR-200c/141 promoter region ( Fig. 8c ). The DNA loop detected using the anchor 1 brings together the 5′-end sequences of miR-200c/141 and the PTPN6 promoter regions. This interaction was further validated by the use of a reciprocal primer (anchor 2) located in the PTPN6 promoter ( Fig. 8d ). Using anchor 2, we observed that PTPN6 promoter not only interacts with miR-200c/141 promoter, but also with a large genomic locus of ∼ 10 kilobases in length. This locus includes the PTPN6 3′-extremity, the miR-200c/141 promoter region and a region downstream from the miRNAs that reaches the 3′-end of the PHB2 gene ( Fig. 8d ). Thus, PTPN6 gene is organized in a 3D gene-loop-like structure, which includes the PTPN6 promoter and its 3′-extremity but also the miR-200c/141 locus. In SKOV3 cells, characterized by low levels of pri-PTPN6 and pri-miR-200c/141 transcripts, the physical interaction between the two promoters was undetectable with the primer anchor 1 ( Fig. 8e ). Similarly, using the primer anchor 2, the interaction frequency between PTPN6 and miR-141/200c promoters was close to background ( Fig. 8f ). Although the PTPN6 intragenic-loop (bringing together PTPN6 5′- and 3′-ends) was still detected, it did not include the large downstream region containing the miR-200c/141 gene ( Fig. 8f ). Moreover, although detectable, the interaction between PTPN6 5′- and 3′-ends was lower in SKOV3 than in IGROV-1 cells ( Fig. 8d,f ). This was expected as intragenic DNA loops have already been associated with transcriptional activity [50] , [55] . Altogether, these observations suggest that high-level expression of both PTPN6 and miR-200c/141 genes is associated with the formation of a 3D DNA loop associating their respective promoters. Still, the upregulation of both PTPN6 and pri-miR-200c-141 transcription by H 2 O 2 treatment in SKOV3 cells was not enough to induce a detectable change in the 3D conformation ( Fig. 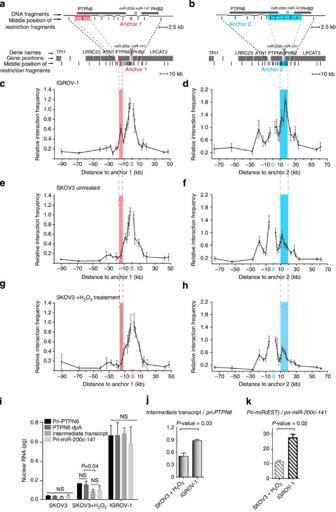8g,h ). Figure 8:PTPN6andmiR-200c/141promoters interact with each other through a DNA loop. (a,b) Schematic representations ofmiR-200c/141genomic locus, DNA fragments generated by chromatin digestion and anchors 1 (a) and 2 (b) used for 3C experiments. On the bottom part, genes surroundingmiR-200c/141-coding region are shown as grey boxes. Each vertical line, indicated beneath boxes, corresponds to the middle position of each restriction fragment analysed. The upper parts of the schemas are high magnification ofPTPN6-miR-200c-141-PHB2genomic locus. Black arrows indicate the sense ofPTPN6andPHB2transcription. DNA restriction fragments, generated by chromatin digestion usingNcoI restriction enzyme, are indicated by horizontal lines. Each vertical line, beneath the fragments, shows the middle position of each restriction fragment analysed. Are also indicated the positions of anchors 1 and 2 inmiR-200c/141promoter (a) andPTPN6promoter (b), respectively. The red and blue shaded areas correspond to the genomic regions that interact with anchors 1 and 2, respectively. (c,d) 3C experiments from IGROV-1 ovarian cancer cells. The curves represent the relative interaction frequency of each DNA fragment with anchors 1 (c) and 2 (d), respectively.Xaxis represents the genomic distances from the anchor. Values are means±s.e.m.n=4 independent experiments. (e,f) 3C experiments from SKOV3 ovarian cancer cells. (g,h) 3C experiments from SKOV3 cell line exposed during 3 h to H2O2treatment. (i) Quantity of each RNA entity detected alongPTPN6andmiR-200c-141genomic locus (pri-PTPN6, PTPN6dpA, intermediate and pri-miR-200c-141 primary transcripts), assessed by qPCR using cDNA from nuclear RNA of untreated SKOV3 cells, H2O2-treated SKOV3 cells and in IGROV-1 cells, as indicated. Quantifications were assessed using the standard curves shown in (Supplementary Fig.6a). Quantities are expressed in picogram (pg). (j,k) Ratios of quantities of Intermediate transcript versuspri-PTPN6primary transcript andpri-miR(EST)versuspri-miR-200c-141transcript in SKOV3+H2O2and IGROV-1 cells. Data are means of±s.e.m.n=6 independent experiments per cell line.P-values are from Student’st-test. NS, not significant. Figure 8: PTPN6 and miR-200c/141 promoters interact with each other through a DNA loop. ( a , b ) Schematic representations of miR-200c/141 genomic locus, DNA fragments generated by chromatin digestion and anchors 1 ( a ) and 2 ( b ) used for 3C experiments. On the bottom part, genes surrounding miR-200c/141 -coding region are shown as grey boxes. Each vertical line, indicated beneath boxes, corresponds to the middle position of each restriction fragment analysed. The upper parts of the schemas are high magnification of PTPN6-miR-200c-141-PHB2 genomic locus. Black arrows indicate the sense of PTPN6 and PHB2 transcription. DNA restriction fragments, generated by chromatin digestion using Nco I restriction enzyme, are indicated by horizontal lines. Each vertical line, beneath the fragments, shows the middle position of each restriction fragment analysed. Are also indicated the positions of anchors 1 and 2 in miR-200c/141 promoter ( a ) and PTPN6 promoter ( b ), respectively. The red and blue shaded areas correspond to the genomic regions that interact with anchors 1 and 2, respectively. ( c , d ) 3C experiments from IGROV-1 ovarian cancer cells. The curves represent the relative interaction frequency of each DNA fragment with anchors 1 ( c ) and 2 ( d ), respectively. X axis represents the genomic distances from the anchor. Values are means±s.e.m. n =4 independent experiments. ( e , f ) 3C experiments from SKOV3 ovarian cancer cells. ( g , h ) 3C experiments from SKOV3 cell line exposed during 3 h to H 2 O 2 treatment. ( i ) Quantity of each RNA entity detected along PTPN6 and miR-200c-141 genomic locus (pri-PTPN6, PTPN6dpA, intermediate and pri-miR-200c-141 primary transcripts), assessed by qPCR using cDNA from nuclear RNA of untreated SKOV3 cells, H 2 O 2 -treated SKOV3 cells and in IGROV-1 cells, as indicated. Quantifications were assessed using the standard curves shown in ( Supplementary Fig.6a ). Quantities are expressed in picogram (pg). ( j , k ) Ratios of quantities of Intermediate transcript versus pri-PTPN6 primary transcript and pri-miR(EST) versus pri-miR-200c-141 transcript in SKOV3+H 2 O 2 and IGROV-1 cells. Data are means of±s.e.m. n =6 independent experiments per cell line. P -values are from Student’s t -test. NS, not significant. Full size image DNA loop is associated with increased read-through Finally, we investigated whether the DNA loop observed between the PTPN6 and miR-200c/141 promoters in IGROV-1 cells could favour the read-through from the PTPN6 gene. To do so, we compared PTPN6 primary transcript levels with that of the intermediate transcript in IGROV-1 and SKOV3 cells upon stress ( Fig. 8i,j and Supplementary Fig. 5c for RT-negative controls). The ratio between intermediate transcript and PTPN6 primary transcript levels was of 1 in IGROV-1 cell line, whereas of 0.56 in SKOV3 upon stress, indicating that the DNA loop is associated with increased read-through ( Fig. 8j ). In both SKOV3 and IGROV-1 cells, the levels of the different transcripts detected along the intermediate region and the pri - miR-200c-141 genomic locus were equivalent among them ( Fig. 8i ). This means that independently of PTPN6 transcription initiation rate and percentage of bypass, each molecule of the PTPN6 bypassed transcript corresponds to one molecule of pri-miR-200c-141 primary transcript, indicating a major role of the read-through. We also analysed the different quantities of the pri-miR-200c-141 primary transcript (intronic isoform) with this one of the exonic isoform, corresponding to previously described ESTs (referred to as pri-miR(EST), see Fig. 5a for genomic localization). Globally, the quantity detected of pri-miR(EST) was at least tenfold higher than pri-miR-200c-141 primary transcript (intronic isoform), most probably because pri-miR(EST) is stabilized and/or submitted to additive regulation. Here again, we observed that the differential expression between the two cell lines was maintained and 2.4-times higher in IGROV-1 than in SKOV3+H 2 O 2 cells ( Fig. 8k ). Taken as a whole, our work shows that the 3D DNA loop linking PTPN6- and miR-200c/141 -specific promoters contributes, with the transcriptional bypass of the PTPN6 polyadenylation site, to the fine co-regulation of these two transcript units ( Fig. 9 ). We provide here evidence that intergenic miRNAs can be regulated through a transcriptional read-through and a 3D chromatin interaction between different promoters. The miR-200 family members exhibit key roles in oxidative stress response and ovarian tumorigenesis, oxidative stress being also an important feature of HGSOC [2] , [4] , [5] , [7] , [9] , [10] , [32] . Understanding the mechanisms involved in their regulation is an important question to highlight new insights of their functions in these patho-physiological conditions, especially in the characterization of ovarian cancer molecular subgroups. Here, we demonstrate that the transcription rate of the miR-200c/141 transcription unit is a crucial step in determining mature miRNAs levels within cells, both at basal state and upon stress. Moreover, we unravel two original and complementary mechanisms by which the transcription of miR-200c/141 is regulated: a transcriptional read-through of an upstream gene, PTPN6, and a transcription co-regulation mediated through a 3D DNA loop linking the two closely located PTPN6 and miR-200c/141 promoters. Data from the last decade demonstrated that chromatin conformation is not randomly determined and has important roles in gene regulation. Studies in yeast have shown that DNA loops linking promoter and terminator regions of the same gene are important for transcriptional memory and directionality [56] . Examples of such 3D DNA conformation have also been described in humans and were associated with transcriptional repression [56] , [57] , [58] . Our data uncover a new example of such short-range chromatin interaction in human cells that can participate in miRNA regulation. Indeed, we highlight here a chromatin interaction that brings close together the promoters of PTPN6 and miR-200c/141 genes. Importantly, the chromatin loop we discovered between these two transcription units ( PTPN6 and miR-200c/141 ) does not correspond to the gene-loops previously described between the promoter and terminator regions within the same gene [58] , [59] , [60] . In contrast to these intragenic DNA loops, the chromatin loop we uncovered extends from the PTPN6 promoter to a region far downstream of the PTPN6 3′-end, reaching the miR-200c/141 promoter and spanning at least 10 kilobases. Interestingly, we also detected that the promoter region of the ATN1 -encoding gene, located upstream PTPN6 may also interact with PTPN6 and be another partner in the fine regulation of this genomic locus. The interaction between 5′-end of PTPN6 and miR promoter could facilitate the RNA polymerase II recycling from the PTPN6 3′-end to its start site, as well as from the pri-miR-200c-141 3′-end to the PTPN6 start site. Given the strict correlation of transcription between these two genes, we propose that the physical association of the two promoters plays a positive role in their co-regulation. Consistent with this idea, the formation of this 3D DNA loop is linked to the expression rates of the two genes and the proportion of read-through from the PTPN6 gene. Although the 3D DNA structure is formed in cells with high basal levels of expression of the two genes, it remains undetected in cells with a low basal expression rate. Accordingly, the levels of DNA methylation and active histone marks, such as H3K9Ac and H3K4me3, are tightly equivalent between PTPN6 and miR-200c/141 promoters. Some of the epigenetic silencing marks could be reversible and removed by oxidative stress. Our results are in agreement with previous studies showing that in breast, lung, colon, bladder and prostate cancer cells, miR-200c/141 levels are consistent with DNA methylation status and histone modifications detected in their promoter regions. We confirmed these results in ovarian cancer cells and extended them to the promoter of the upstream and co-regulated gene, PTPN6 . Finally, we demonstrate here that the 3D DNA loop is associated with a 2.5-fold increase in transcription read-through from the upstream gene, PTPN6 . It is important to note that given the physical interaction between the two promoters that we demonstrated here, the crosslink between the promoters could also contribute to the ChIP experiments results. Nevertheless, our results are consistent with the fact that both genes could be under equivalent epigenetic regulation, which is in complete agreement with the coordinated epigenetic and transcriptional regulation of these genes. In addition to the DNA loop, our data unravel the read-through from the PTPN6 gene, as another original mechanism linking PTPN6 and miR-200c/141 genes. Indeed, we demonstrate the existence of an intermediate transcript extending from the 3′-end of the PTPN6 gene to the miR-200c/141 transcription unit. It is mediated through the transcriptional bypass of the usual PTPN6 polyA site, allowing the RNA polymerase II to reach the downstream miR-200c/141 transcription unit. We identified two downstream APA sites used for the termination of the pri-miR-200c-141 primary transcript. The first corresponds to the already established ESTs, located downstream of the miR-200c/141 genomic sequences. The second APA site, located very close to the PHB2 polyadenylation signal, is conserved between human and mouse species and had not been reported previously ( Supplementary Fig. 5 ). One should note, however, that the polyadenylation of the PTPN6 transcripts at these APA sites is not necessarily required for the production of the miRNAs in the same round of PTPN6 transcription. Indeed, miRNAs can be processed by Drosha co-transcriptionally and a late termination of RNA Pol II polymerization downstream from the PTPN6 3′-end can be sufficient for the transcription of the downstream miR-200c/141, even when PTPN6 mRNA is polyadenylated at its usual site. Such regulation of intergenic miRNAs through upstream transcription has been postulated by Proudfoot and colleagues [61] . We give here, for the first time, evidence of this type of miRNA transcription. We have investigated to which extent each of these two mechanisms (DNA loop versus PTPN6 read-through) contributes to miR-200c/141 primary transcription. The pri-miR-200c-141 levels being the result of both PTPN6 read-through and independent transcription initiation, we have carefully assessed the quantity of the different primary transcripts detected along PTPN6 and miR-200c/141 genomic locus. We observed that the read-through from the PTPN6 gene is a dominant mechanism in ovarian cancer cells, each molecule of the pri-miR-200c-141 primary transcript corresponding to one molecule of bypassed PTPN6 polyadenylation signal. Thus, the transcriptional PTPN6 read-through could be the major mechanism explaining the strikingly similar kinetics of PTPN6 and pri-miR-200c-141 upregulation following stress. Ideally, to demonstrate the impact of the PTPN6 gene on pri-miR-200c-141 transcription, a homozygous genetic knock-out model of the PTPN6 gene would be required to definitely prove the role of PTPN6 transcription on miR-200c/141 regulation. A natural mutated mouse model for Ptpn6 exists, the motheaten mice, but as the Ptpn6 transcription is not impaired in these mice, they are not appropriate to investigate this question. We have thus evaluated if the read-through from the PTPN6 gene can influence miR-200c-141 transcription, by using the CRISPR/Cas9 technology. Deletion of PTPN6 promoter demonstrated that PTPN6 transcription is required for miR-200c-141 primary transcription in SKOV3 cells. Unfortunately, PTPN6 silencing is deleterious for the survival of IGROV-1 cells, characterized by high basal PTPN6 expression rate. Being detected in cells with high expression levels, we can speculate that the 3D chromatin structure and subsequent high interaction frequency between the two promoters favours the co-regulated transcription of the two genes. The read-through molecule can reach the miRNAs locus, as demonstrated previously, or also favour the start of the polymerization from the miR-200c/141 TSS. In contrast, in cell lines that exhibit low basal expression rate of PTPN6 and miR-200c/141 , such as SKOV3, the interaction frequency between the two promoters is low. Interestingly, our data suggest also that the 3D DNA loop is not only associated with a high rate of transcription initiation but also of read-through from the PTPN6 gene. The so finely regulated co-expression of PTPN6 and miR-200c/141 suggest a functional relationship between the two genes. The levels of the miR-200 family members are reproducibly upregulated upon oxidative stress conditions in various cell lines and participate in stress response. Interestingly, the co-regulated gene PTPN6 encodes for a Protein Tyrosine Phosphatase that is itself implicated in anti-oxidant defense [62] . Importantly, in HGSOC, the oxidative stress signature has a prognostic value and the miR-200s are significantly upregulated, as shown by several independent studies [2] , [4] , [5] , [7] , [32] . In that sense, our data on the mechanism of their regulation give another additive insight into the different ovarian transcriptomic subgroups defined by the miR-200/141. In complete agreement with our results, PTPN6 is also generally overexpressed in ovarian cancer cells and in HGSOC [63] , [64] , [65] . PTPN6 and miR-200s play a physiological role in oxidative stress regulation and interestingly, they have both a negative impact on the p38 pathway. Indeed, in cells depleted for PTPN6 , the levels of phosphorylated p38 are increased [66] . The activation of this key redox sensor that is also directly targeted by miR-14/200a (ref. 7 ) is rescued by a treatment with an antioxidant [66] . Finally, the 3C experiment also revealed that the promoter of the ATN1 gene, located upstream PTPN6 , could interact with PTPN6 5′-end. As ATN1 is involved in OXPHOS regulation and mitochondrial disorders [67] , this observation may represent interesting new clues for the global regulation of this genomic locus by oxidative stress, and for its role in this process. These results are complementary to previous studies [68] showing a reciprocal interaction between miRNA and their regulatory transcription factor. Indeed, one of the largest known mammalian miRNA-containing cluster, Gtl2-Dio3, is regulated by MEF2A, a key transcription factor involved in skeletal muscle. Reciprocally, these miRNA directly target the secreted Fizzled-related protein 2, an inhibitor of the wingless-type (WNT) pathway. These observations are similar to our own findings showing the co-regulation of PTPN6 and miR-200c/141 by oxidative stress, the two exerting a role in oxidative stress response. Altogether, these data give complementary insights of the interplay between miRNA, their regulatory elements and the processes in which they are involved. The kind of transcriptional regulation we describe here are probably not restricted to these miRNAs and other examples of such mechanisms are likely to be discovered in the future. Cell culture and treatments All cells lines were cultured in DMEM (Invitrogen, # 41966) supplemented with 10% fetal bovine serum (except for immortalized mouse fibroblasts, which were maintained in 7% fetal bovine serum) at 37 °C and 5% CO 2 atmosphere. Cells were treated with hydrogen peroxide, H 2 O 2 (400 μM), except WI38 treated with 200 μM H 2 O 2 , for different periods of time, as indicated on each figure (up to 8 h). H 2 O 2 was purchased from Sigma (#H-1009) and dilutions in H 2 O were prepared just before use. Mouse fibroblast cells were submitted for 3 h to various stresses increasing ROS levels: 50 μM menadine sodium bisulfite (Sigma, #M2518), 200 μM Arsenic (Sigma, #35000), 300 mM Sorbitol (Sigma, #85529). To inhibit transcription, cells were treated with 5 μM actinomycin D (Sigma, #A9415) during 4 h. The DNA-demethylating agent 5-Aza-2′-deoxycytidine (Sigma, #A3656) was diluted in dimethylsulphoxide and added to the cells at a final concentration of 10 μM. Medium was changed after 48 h and cells were treated for 96 h before lysis. RNA extraction Total RNA isolation was performed using miRNEasy Kit from (Qiagen, #217004) according to the manufacturer’s instructions. RNA concentrations were determined with a NanoDrop apparatus (NanoDrop Technologies, Inc.), and RNA integrity was verified using Agilent RNA 6000 Nano Kit (Agilent, #5067–1511) and apparatus. Before complementary DNA synthesis, RNA were treated with DNaseI, RNase free (Thermo Scientific, #EN0525) in reaction buffer with MgCl 2 according to the manufacturer’s protocol. Nuclear RNA extraction Cells were resuspended in nuclear extraction buffer (Tris 10 mM pH 7.5; 10 mM NaCl; 5 mM MgCl 2 ; 0.5% NP-40), incubated at 4 °C for 5 min and spin down 5 min at 500 g . The cytosolic fraction was discarded. The pellet, corresponding to the nuclear fraction, was washed twice in the nuclear extraction buffer, resuspended in Trizol and passed through a 20-G needle five times. RNA extraction was done with mi-RNeasy kit (QIAGEN #217004) and RNA concentrations were determined with a NanoDrop apparatus (NanoDrop Technologies, Inc.). Before cDNA synthesis, nuclear RNA were treated with DNaseI, RNase free (Thermo Scientific #EN0525) in reaction buffer with MgCl 2 according to the manufacturer’s protocol. Real-time reverse transcription (RT)–PCR Primary transcripts and mRNAs levels were assessed using SYBR qRT–PCR assay. Reverse transcriptase reactions were performed using 1 μg of DNAse-treated total RNA per sample and iScript RT Kit (Bio-Rad, #170–8897) or SuperScript III Reverse Transcriptase with oligo(dT) and random primers (Invitrogen, #180 80–051). SYBR Power master mix (Applied Biosystems, #4367659) was used for qPCR with primers at 300 nM final concentration each. GAPDH, U6 snRNA and CYCLOPHYLIN B were used as loading controls. TaqMan qRT–PCR assay was used for detection of mature miRNAs. Reagents, primers and probes were obtained from Applied Biosystems. RT reactions and real-time qPCR were performed according to manufacturer protocols from 50 ng of RNA per sample. Primers and probes are specific for each miRNA and are designed by the manufacturer. U6 snRNA and miR-16 were used as loading controls. qPCR reactions were performed in a Chromo4 apparatus (Bio-Rad). Relative expression was calculated using the comparative cycle threshold method (2 ΔΔCt ) and the Opticom Monitor 3 software. qPCR primers were designed using PrimerQuest (Integrated DNA Technologies) and were purchased from Sigma. The efficiency of each couple of primer used for qPCR was verified using serial dilutions of the template. When comparing transcript levels between different couples of primers, normalization using standard DNA was performed. Normalization was done using control DNA template obtained from the RP11-8J11 BAC clone (bacpac.chori.org), containing PTPN6 and miR-200c/141 genomic region. For each primer pair, quantification was performed using the coefficients from the standard curve calculated using the control template dilutions measured in the same qPCR plate. Schematic representation of the genomic positions of the primers is indicated in Fig. 5a and sequences are given in Supplementary Table 2 . RT–PCR reactions using Set 2 and Set 3 primers were performed on cDNA from cells and HGSOC using Phusion DNA Polymerase (Thermo Scientific, # F-530) according to the manufacturer’s instructions and with the GC buffer. During the first ten cycles of the PCR reactions, the annealing temperature increased 0.5 °C every cycle, from 60° to 65 °C and was maintained at 65 °C for the following cycles. The reactions were stopped after either 25, 30, 35 or 40 cycles. The PCR products were loaded on 0.8% agarose gel then transferred onto Hybond N+ membrane (GE Healthcare, # RPN203B). Membranes were hybridized with γ-ATP 32 P-labelled primers (5′-TGACCCTGTATATAGCCCAGCCA-3′ and 5′-AGCAAACAAAGCCTGGGAGAGAGA-3′) in ULTRAhyb Ultrasensitive Hybridization Buffer (Ambion, # AM8669). Signals were detected with Typhoon and quantified with Multi Gauge software. All primer sequences used for PCR and qPCR are given in Supplementary Table 2 . Amplified bands were purified, cloned in TA-vector (Invitrogen#45.0030) and submitted to sequencing in order to verify that they corresponded to the expected intermediate transcript sequence. CRISPR/Cas9 experiment Target-specific CRISPR guide RNAs (sgRNA) were designed by GeneCoppeia to have limited off-targets. Corresponding primers were subcloned into the All-in-one sgRNA plasmid (GeneCopoeia, #CS-HCP000300-2-CG01-1-LR). The sequences flanking PTPN6 promoter region targeted by the CRISPR guide RNAs are: sgRNA1: 5′-GATAACGCCTGCAACGACAT-3′; sgRNA2: 5′-GCCTGCCACCCACGGTAGAC-3′. Twenty-four hours before transfection, 5 × 10 5 SKOV3 cells were seeded into six-well plates. Cells were transfected using Cell Avalanche Transfection Reagent (EZ-Biosystems #EZT-IGRO-1), provided by the company for enhancing transfection efficiency in IGROV-1 Ovarian cancer cells, but which also improved significantly the transfection efficiency in SKOV3 cell line. Three micrograms of sgRNA-recombined vector (containing the sgRNA1 and sgRNA2) were transfected using the manufacturer’s protocol. Twenty-four hours post transfection, the cells were transiently selected (for 24 h) with hygromycine B Gold (InvivoGen, #ant-hg-1) in order to eliminate non-transfected cells. Transfection protocol was repeated four times on total cell populations. Sixty-three individual clones were next isolated by limited dilution and analysed at genomic level. PCR- and qPCR-based genotyping methods were used to identify the clones in which the genomic deletion occurs and to quantify the DNA copy number of the targeted region relative to control regions, measuring the efficiency of CRISPR deletion as creating allelic deletions, SKOV3 cells being tetraploid. Sequences of the primers used for the genotyping were designed either inside or outside the targeted region, as schematically represented in Fig. 6a . Sequences of the primers are given in Supplementary Table 2 . Genomic DNA of the 60 individual clones was purified with DNAeasy blood and tissue kit (Qiagen, #69504) using the manufacturer’s instructions. qPCR was performed with 50 ng of genomic DNA in duplicate using SYBR green master mix (Roche) on a Chromo4 apparatus (Bio-Rad). Relative levels of DNA copy number were calculated using the 2 ΔΔCt method with copy number normalized to glyceraldehyde-3-phosphate dehydrogenase (GAPDH) intron 1 (chromosome 12) as a control. Two individual clones exhibited a significant reduction of DNA copy number in the targeted region, with two- and three-recombined alleles among four, respectively. To obtain complete deletion of the four alleles, these two individual clones were submitted to two additive rounds of transfections and re-analysed at genomic level, using the same PCR- and qPCR-based genotyping method, as described above. Two clones referred to as SKOV3-Δ1 and SKOV3-Δ2 exhibited tetra-allelic recombination and deletion of the PTPN6 promoter-targeted region and were considered for further analyses. The amplified fragments from genotyping PCR and qPCR have been isolated, cloned and sequenced to verify that they correspond to the recombined PTPN6 genomic locus after deletion. HGSOC cohorts The Institut Curie cohort is described in ref. 7 . Analyses based on the Curie cohort were approved by the Institutional Review Board and Ethics committee. Before inclusion in the study, patients were informed that their biological samples could be used for research purposes and that they had the right to refuse if they wished so. Analysis of tumour samples was performed according to the relevant national law on the protection of people taking part in biomedical research. Only samples enriched in at least 65–70% epithelial cells have been considered in our study. miRNA and mRNA levels were assessed by qPCR using TaqMan and SYBR assays as described in ref. 7 . Microarray data are accessible in the Gene Expression Omibus under the accession number GSE26193. All the data from the TCGA cohort was obtained from the TCGA Data Portal ( https://tcga-data.nci.nih.gov/tcga/ ). Patient characteristics and clinical features of the two cohorts analysed in our study are listed in Supplementary Table 1 , in order to facilitate their comparison. TCGA data are provided from tumour samples with at least 60% of enrichment in epithelial tumour cells, as mentioned in the Supplementary Information in ref. 51 . Copy number analyses in ovarian cancer samples For the Curie cohort, SNP 100K data were analysed using Partek Software. Raw data were imported into Partek using default parameters and the Partek baseline for copy number calculation, followed by a GC-adjustment. The segmentation parameters used were 15 markers, a signal-to-noise ratio of 0.3 and a P -value of 0.001. The threshold used for defining amplified/deleted patients in the PTPN6 and miR-200c/141 region was ±0.3. For the TCGA cohort, copy number data were downloaded from: https://tcga-data.nci.nih.gov/tcga/ (Level 3 data, MSKCC 1x1M-G447A). Data were imported and analysed using R version 2.12.2. Segments defined in TCGA data were used to classify unchanged, amplified or deleted patients in the region of interest. The classification was made according to segment mean values in a window of 150 kb in the chromosome 12p13 including PTPN6 and miR-200c/141 . Patients were considered as ‘Amplified’ or ‘Deleted’, if any segment mean value in this region was above +0.3 or below −0.3, respectively. ‘Unchanged’ patients were those who exhibit neither amplifications nor deletions in the region of interest, according to this threshold. TCS analyses TCS were computed as described in ref. 52 . Briefly, from the microarray data, a list containing only one probeset per gene is made. Next, for each gene, the TCS is computed as the sum of the correlation coefficients (Spearman’s rho coefficient) between the gene and its 2n neighbours ( n =10). To define a significance threshold ( P =0.001), TCS were computed using randomized positions for probesets and the TCS of the 1,000th quantile was used. For the TCS Maps, TCS values of each gene are plotted against the corresponding genomic position. NCI-60 and Sanger Cell Line Project data sets For the NCI-60 panel, Agilent microarray data were obtained from CellMiner Database ( http://discover.nci.nih.gov/cellminer/loadDownload.do ) and miRNA qPCR data were obtained from the Israel lab http://dtp.nci.nih.gov/mtargets/download.html . For the Sanger Cell Line Project panel, microarray data were obtained from the Broad Institute website ( http://www.broadinstitute.org/cgi-bin/cancer/publications/pub_paper.cgi?mode=view&paper_id=189 ). Affymetrix Plus 2.0 probeset 206687_s_at was used for PTPN6 levels. All the non-haematopoietic cell lines were included in the analyses. Methylated DNA Immunoprecipitation MeDIP experiments were performed using MagMEDIP kit from Diagenode (#C02010020), according to the manufacturer’s instructions. Briefly, genomic DNA was extracted from 3 to 10 million cells and sonicated using the Bioruptor apparatus (Diagenode) to obtain fragments of 100–600 bp in length (10 min at ‘low’ power with cycles of 15 s ON and 15 s OFF). For each reaction, 1 μg DNA was used. Positive (methylated DNA) and negative (unmethylated DNA) controls were added to the reaction, in order to normalize for the immunoprecipitation (IP) efficiency. IP using anti-5-methylcytosine antibody and magnetic beads was performed overnight at 4 °C. After washing and elution, immunoprecipitated DNA was measured by qPCR and reported to input DNA. Chromatin immunoprecipitation Cells were crosslinked for 15 min using formaldehyde (1% final concentration) (Sigma, #F8775) at room temperature. Next, they were harvested and nuclei were extracted, lysed and sonicated. IP was performed using magnetic beads (Invitrogen, #100-02D) and 5 μg of antibody for each condition. Anti-RNA Polymerase II antibody was purchased from Santa Cruz (sc-899) and histone antibodies were purchased from Abcam: H3K4me3 (ab8580), H3K9Ac (ab10812), H3 (ab1791). After reverse crosslink, ChIP enriched fragments were evaluated by qPCR and reported to input DNA levels. Chromosome conformation capture 3C experiments were performed based on protocols previously established [69] with modifications. Fifty million cells were crosslinked with 2% formaldehyde for 10 min at room temperature and lysed in the following buffer: 10 mM Tris-Cl, pH 8.0; 10 mM NaCl; Igepal (NP-40), 0.2% (v/v) containing protease inhibitors. DNA was digested overnight with the restriction enzyme Nco I (New England BioLabs) in a buffer containing final concentration of 1% Triton X-100 and 0.1% SDS. The restriction enzyme was chosen in order to investigate the short-range chromatin interaction with a high-resolution capacity in our region of interest. Ligation in diluted conditions (total of 80 ml) was performed at 16 °C for 4 h followed by 30 min at room temperature using T4 ligase from Promega (# M1794). After overnight reverse crosslink at 65 °C with proteinase K (Roche, #03 115 836 001), DNA was extracted with phenol and chloroform and precipitated in ethanol. RNAse (Roche, #11 119 915 001) treatment was performed followed by supplementary phenol chloroform extractions and ethanol precipitation. For each experiment, purity of 3C template was assessed as described in ref. 69 . Restriction efficiency at each Nco I site was calculated from non-ligated controls and was of 60–70% in average. Primer normalization was done using control template obtained from digestion and ligation of the RP11-8J11 BAC clone (bacpac.chori.org). For each primer pair, quantification was performed using the coefficients from the standard curve calculated using the control template dilutions measured in the same qPCR plate. For each fragment, a relative interaction frequency over the first 3′ fragment from the anchor was computed (by dividing the interaction frequency of a given fragment to this one of the closest 3′-fragment from the anchor) and plotted according to its distance to the anchor. All primers and modified probes were purchased from MGW Operon. Primer and anchor (probes) sequences are given in Supplementary Table 3 . 3′ and 5′ RACE RACE experiments were performed using the RLM-RACE kit from Ambion (#AM 1700) according to the manufacturer’s instructions. The 5′ RACE protocol is designed to detect only capped mRNA. Primers used for RACE experiments are listed in Supplementary Table 2 . ZEB1, ZEB2 or TP53 silencing 2 × 10 5 SKOV3 and IGROV-1 cells were transfected the day after seeding with 10 nM of each siRNA using Dharmafect 1 transfection reagent (Dharmacon, T-2001) according to the supplier’s recommendations. Forty-eight hours post transfection, SKOV3 cells were either untreated or treated with 400 μM H 2 O 2 for 1 h before RNA extraction and purification using miRNeasy kit from Qiagen. mRNA levels were measured using SYBR RT–qPCR (see above) with specific primers. GAPDH was used for internal control of mRNA quantity. SKOV3 cells are TP53 null and no expression of ZEB2 was detected in IGROV-1 cell line, thus SKOV3 and IGROV-1 were not silenced using TP53- and ZEB2 -specific siRNA, respectively. siRNA used for transfection were: siZEB1 (smart pool from Dharmacon #L-006564); siZEB2 (smart pool from Dharmacon #L-006914); siTP53 (smart pool from Dharmacon #L-003329) and siCtl (Control; Dharmacon #D-001810-01). Primer sequences used for qPCR are given in Supplementary Table 2 . Statistic analyses and databases Data are generally reported as means±s.e.m. (or s.d. when specified), obtained from at least three independent experiments, using adapted statistical test, as mentioned. Correlation coefficients are indicated by ρ (rho) and correspond to Spearman’s rank correlation coefficients. The genome sequence data were obtained from University of California at Santa Cruz (genome.ucsc.edu). How to cite this article: Batista, L. et al. Regulation of miR-200c/141 expression by intergenic DNA-looping and transcriptional read-through. Nat. Commun. 7:8959 doi: 10.1038/ncomms9959 (2016).